Gross violation of the Wiedemann–Franz law in a quasi-one-dimensional conductor When charge carriers are spatially confined to one dimension, conventional Fermi-liquid theory breaks down. In such Tomonaga–Luttinger liquids, quasiparticles are replaced by distinct collective excitations of spin and charge that propagate independently with different velocities. Although evidence for spin–charge separation exists, no bulk low-energy probe has yet been able to distinguish successfully between Tomonaga–Luttinger and Fermi-liquid physics. Here we show experimentally that the ratio of the thermal and electrical Hall conductivities in the metallic phase of quasi-one-dimensional Li 0.9 Mo 6 O 17 diverges with decreasing temperature, reaching a value five orders of magnitude larger than that found in conventional metals. Both the temperature dependence and magnitude of this ratio are consistent with Tomonaga–Luttinger liquid theory. Such a dramatic manifestation of spin–charge separation in a bulk three-dimensional solid offers a unique opportunity to explore how the fermionic quasiparticle picture recovers, and over what time scale, when coupling to a second or third dimension is restored. The success of Fermi-liquid (FL) theory in describing the properties of most ordinary three-dimensional metals makes it one of the triumphs of twentieth-century theoretical physics. Its wide-ranging applicability is testament to the validity of describing a system of interacting electrons by mapping its low-lying quasiparticle excitations onto a Fermi gas of non-interacting electrons. Perhaps the most striking realization of this one-to-one correspondence is the validity of the Wiedemann–Franz (WF) law in almost all known theoretical [1] , [2] , [3] , [4] and experimental [5] , [6] , [7] cases. The WF law states that the ratio of the electronic thermal conductivity κ e to the electrical conductivity σ at a given temperature T is equal to a constant called the Lorenz number or Lorenz ratio, L 0 = κ e / σT =( π 2 /3)( k B / e ) 2 and reflects the fact that thermal and electrical currents are carried by the same fermionic quasiparticles. Although the WF law is most applicable in the zero temperature (impurity scattering) limit, it is found to hold equally well at room temperature once all inelastic scattering processes become active [8] . A marked deviation from the WF law is theoretically predicted when electrons are spatially confined to a single dimension. In systems that are strictly one-dimensional (1D), even weak interactions destroy the single particle FL picture in favour of an exotic Tomonaga–Luttinger liquid (TLL) state in which the fundamental excitations are independent collective modes of spin and charge, referred to, respectively, as spinons and holons. As heat is transported by entropy (spin and charge) and electric current by charge alone, spin–charge separation is a viable mechanism for the violation of the WF law [9] , [10] , [11] , [12] . Physically, repulsive interactions in a disordered 1D chain can inhibit the propagation of holons relative to that of spinons, leading to a strongly renormalized Lorenz number [9] . Experimental signatures of TLL physics have been seen in the spectral response of a number of 1D structures [13] , [14] , [15] and bulk crystalline solids [16] , [17] , [18] , [19] , [20] . Although the ratio κ e / σT can in principle provide a direct means of distinguishing between FL and TLL states at low energies, there have been no confirmed reports to date of WF law violation in any 1D conductor. Identifying such systems, particularly bulk systems, is important as it might then allow one to tune, chemically or otherwise, the effective interchain coupling and thereby drive the system from one electronic state to the other. This would then open up the possibility of exploring the TLL-to-FL crossover and the nature of the excitations in the crossover regime. Here we report a study of the electrical and thermal conductivity tensors of the purple bronze Li 0.9 Mo 6 O 17 , a quasi-1D conductor whose (surface-derived) photoemission lineshapes [19] , and density of states profiles [20] contain features consistent with TLL theory. 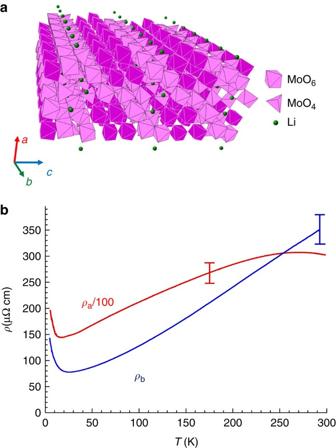Figure 1: Crystal structure and electrical resistivity of the quasi-one-dimensional metal Li0.9Mo6O17. (a) Three-dimensional crystal structure showing isolated, conducting, zigzag chains of MoO6octahedra along thebaxis in dark purple and non-conducting octahedra and MoO4tetrahedra in light pink. Li ions are shown as green spheres. (b) Intra-chain (ρb) and inter-chain (ρa) resistivities of Li0.9Mo6O17as a function of temperature. Note thatρahas been scaled by a factor of 1/100. The error bars inρaandρb(±7% and 12%, respectively) represent the uncertainty in the determination of the sample dimensions and the standard deviation of the room temperature resistivity of the subset of curves 1–5 shown with solid lines inSupplementary Figure S1a, respectively. For details of howρbwas determined, please refer to the section on isolating the intrinsic in-chain resistivity in theSupplementary information. Electrical resistivity of Li 0.9 Mo 6 O 17 As shown in Figure 1a , Li 0.9 Mo 6 O 17 possesses a set of weakly coupled zigzag chains of MoO 6 octahedra with a hole-concentration, believed to be close to half-filling [21] , running parallel to the crystallographic b axis. The T -dependence of the b axis resistivity, plotted in Figure 1B , varies linearly with temperature above 100 K, then as T is lowered, ρ b ( T ) becomes superlinear. Below around 20 K, Li 0.9 Mo 6 O 17 undergoes a crossover from metallic to insulating-like behaviour, ascribed to the formation of a putative charge density wave [22] , [23] . Also plotted in Figure 1b is the interchain resistivity ρ a ( T ). The anisotropy in the electrical resistivity, ρ a ∼ 100 ρ b (< ρ c ) agrees well with optical conductivity measurements [24] and highlights the extreme one-dimensionality of the electronic system. Note that although the T -dependence of the resistivity is similar along all three crystallographic axes, the corresponding interchain mean free paths are estimated to be less than the spacing between adjacent zigzag chains, implying incoherent interchain transport, at all finite temperatures. Figure 1: Crystal structure and electrical resistivity of the quasi-one-dimensional metal Li 0.9 Mo 6 O 17 . ( a ) Three-dimensional crystal structure showing isolated, conducting, zigzag chains of MoO 6 octahedra along the b axis in dark purple and non-conducting octahedra and MoO 4 tetrahedra in light pink. Li ions are shown as green spheres. ( b ) Intra-chain ( ρ b ) and inter-chain ( ρ a ) resistivities of Li 0.9 Mo 6 O 17 as a function of temperature. Note that ρ a has been scaled by a factor of 1/100. The error bars in ρ a and ρ b (±7% and 12%, respectively) represent the uncertainty in the determination of the sample dimensions and the standard deviation of the room temperature resistivity of the subset of curves 1–5 shown with solid lines in Supplementary Figure S1a , respectively. For details of how ρ b was determined, please refer to the section on isolating the intrinsic in-chain resistivity in the Supplementary information . Full size image Thermal and electrical Hall conductivities of Li 0.9 Mo 6 O 17 In. most solids, the thermal conductivity κ can be described as the sum of two independent contributions; κ = κ e + κ ph , where κ ph is the phonon thermal conductivity. In metals with short mean-free-paths, these two terms are comparable in magnitude, making it difficult to accurately determine the Lorenz ratio. As shown in the Methods section however, the transverse Hall conductivity κ xy is purely electronic in origin (the phonon current is strictly unaffected by a magnetic field) and thus measurements of the thermal Hall effect (the thermal analogue of the electrical Hall effect) provide a means of isolating the electronic component. Moreover, the ratio of the thermal and electrical Hall conductivities κ xy / σ xy T , known as the Hall Lorenz number L xy , is also expected to be equal to L 0 for a Fermi liquid. In our thermal Hall apparatus (inset to Fig. 2a and described in more detail in the Methods section), a temperature gradient is applied along the conducting chain direction ( b axis, taken here to be the x axis) and a magnetic field H // c ( H // z ) generates a Lorentz force that produces a transverse thermal gradient along a ( y ). 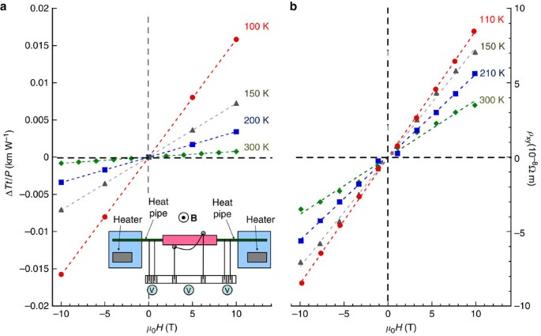Figure 2: Thermal and electrical Hall measurements of Li0.9Mo6O17. (a) Transverse temperature difference ΔTyper unit power (multiplied by the sample thickness) as a function of applied magnetic field at various temperatures. Inset shows a schematic diagram of experimental setup used to measure the thermal Hall effect. Note that the thermocouples were placed either directly opposite to one another or (as shown) displaced longitudinally to allow bothκxxandκxyto be measured simultaneously. Both set-ups gave the same response. ΔTyis dominated by theH-linear, odd-componentκxy. The field-independent component of ΔTydue toκxxhas been subtracted from the data. (b) Hall resistivity as a function of applied magnetic field at various temperatures in the same geometrical arrangement. The main panel in Figure 2a shows the transverse temperature difference Δ T y ( H ), normalized by the applied power and multiplied by the sample thickness, at a number of selected temperatures. As expected, Δ T y is linear and odd in field. Figure 2b shows the electrical Hall resistivity at comparable temperatures. Figure 2: Thermal and electrical Hall measurements of Li 0.9 Mo 6 O 17 . ( a ) Transverse temperature difference Δ T y per unit power (multiplied by the sample thickness) as a function of applied magnetic field at various temperatures. Inset shows a schematic diagram of experimental setup used to measure the thermal Hall effect. Note that the thermocouples were placed either directly opposite to one another or (as shown) displaced longitudinally to allow both κ xx and κ xy to be measured simultaneously. Both set-ups gave the same response. Δ T y is dominated by the H -linear, odd-component κ xy . The field-independent component of Δ T y due to κ xx has been subtracted from the data. ( b ) Hall resistivity as a function of applied magnetic field at various temperatures in the same geometrical arrangement. Full size image To determine κ xy and σ xy at each temperature, it is also necessary to evaluate the longitudinal terms κ xx (= κ b ), κ yy (= κ a ), σ xx (=1/ ρ b ) and σ yy (=1/ ρ a ) (see the Methods section for the derivation of κ xy ). 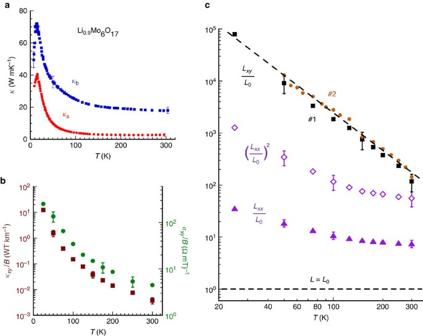Figure 3: The Lorenz ratios of Li0.9Mo6O17. (a) Intra-chain (κb) and inter-chain (κa) thermal conductivities as a function of temperature. The error bars inκ(±15%) represent the uncertainty in the determination of the sample dimensions and the effective distance between the junctions of the differential thermocouple on the sample. (b) Electrical Hall (σxy) and thermal Hall (κxy) conductivities per unit field as a function of temperature. The error bars inσxy(κxy) are estimated from the standard deviation of multiple measurements on different samples. (c) Hall Lorenz ratio (Lxy/L0) for samples no. 1 and no. 2 and the longitudinal Lorenz ratio (Lxx/L0) and its square for no. 1. The error bars inLxy/L0andLxx/L0represent compound errors obtained from the various sources described above. The dotted line is guide to the eye. The horizontal dashed line represents the expectation from Fermi-liquid theory. As shown in Figure 3a , κ a and κ b show marked anisotropy. Due to the extreme resistivity anisotropy, κ a is presumed to be purely phononic in origin and the ab anisotropy in κ ( T ) can be attributed either entirely to the electronic contribution within the chains or to a combination of κ e and additional anisotropy in the phonon spectrum and/or scattering rate. Figure 3: The Lorenz ratios of Li 0.9 Mo 6 O 17 . ( a ) Intra-chain ( κ b ) and inter-chain ( κ a ) thermal conductivities as a function of temperature. The error bars in κ (±15%) represent the uncertainty in the determination of the sample dimensions and the effective distance between the junctions of the differential thermocouple on the sample. ( b ) Electrical Hall ( σ xy ) and thermal Hall ( κ xy ) conductivities per unit field as a function of temperature. The error bars in σ xy ( κ xy ) are estimated from the standard deviation of multiple measurements on different samples. ( c ) Hall Lorenz ratio ( L xy /L 0 ) for samples no. 1 and no. 2 and the longitudinal Lorenz ratio ( L xx /L 0 ) and its square for no. 1. The error bars in L xy /L 0 and L xx /L 0 represent compound errors obtained from the various sources described above. The dotted line is guide to the eye. The horizontal dashed line represents the expectation from Fermi-liquid theory. Full size image Figure 3b shows the resultant thermal and electrical Hall conductivities as obtained from the data presented in Figures 1b , 2a, 2b and 3a . According to the WF law, the ratio κ xy / σ xy should decrease (linearly) with decreasing temperature. In Li 0.9 Mo 6 O 17 , however, the opposite is true; while σ xy increases by a factor ∼ 60 between 300 K and 25 K, κ xy increases by more than 3,000. This implies a change in the Hall Lorenz number L xy (= κ xy / σ xy T ) of more than 500 over the same temperature interval. The thermal Hall angle tan θ T = κ xy / κ e , which provides a measure of the electron mobility, reaches a value ∼ 0.6 at T =50 K and μ 0 H =10 Tesla comparable with that observed in elemental Cu (ref. 25 ). (Here we have assumed that κ e = κ b – κ a ). By comparison, the corresponding electronic Hall angle σ xy / σ xx ∼ 1.25×10 −3 , illustrating the striking difference in mobilities for entropy and charge transport in Li 0.9 Mo 6 O 17 . Lorenz ratios in Li 0.9 Mo 6 O 17 Figure 3c shows L xy / L 0 ( T ) for two samples over the entire temperature range studied. (Note that we have confined our Hall measurements to the metallic regime above the resistivity minimum.) At T= 300 K, L xy / L 0 ∼ 100 and as T falls, L xy / L 0 follows an inverse power-law ∼ T α xy ( α xy ∼ −2.3), reaching a value ∼ 10 5 at T =25 K. The solid triangles in Figure 3c are the corresponding estimates of L xx / L 0 =( κ b – κ a )/ σ b T , that is, assuming an isotropic κ ph . At T= 300 K, L xx / L 0 ∼ 7.5±1.5, rising to ∼ 35 at T =25 K. The horizontal dashed line is the expected FL result. Significantly, in both conventional metals like Cu (ref. 25 ) and Ni (ref. 26 ), and also in correlated metals like YBa 2 Cu 3 O 6.95 (ref. 25 ) and URu 2 Si 2 (ref. 27 ) (whose longitudinal thermal conductivity is dominated by phonons), neither L xx / L 0 nor L xy / L 0 is ever larger than unity. (As shown in Supplementary Figure S1 , we have also verified this result for Ni using our own thermal Hall apparatus). Moreover, according to standard Boltzmann transport theory [26] , L xx / L 0 ∼ <λ s >/<λ e > whereas L xy / L 0 ∼ <λ s > 2 /<λ e > 2 , where <λ s ( e ) > is the Fermi-surface averaged mean free path for entropy (charge) transport, respectively. Hence, in ordinary metals, L xy / L 0 is expected to vary as ( L xx / L 0 ) 2 , as found experimentally [25] . In Li 0.9 Mo 6 O 17 , however, ( L xx / L 0 ) 2 does not scale with L xy / L 0 and cannot be made to scale with L xy / L 0 for any reasonable estimate for the phonon contribution to κ xx ( κ b ). This, together with the unprecedented enhancement of the WF ratio by several orders of magnitude, provides compelling evidence for the breakdown of the conventional FL picture in this quasi-1D conductor. Before discussing the violation of the WF law in Li 0. 9 Mo 6 O 17 in terms of 1D correlation physics, we first consider alternative scenarios based on localization effects. In non-interacting systems, it has been shown theoretically that the WF law is robust to impurity scattering of arbitrary strength up to the Anderson transition [1] , [2] , [3] , [4] . In strongly correlated electron systems, however, the opening of a Mott gap can lead to a strong reduction of the electrical conductivity whereas the transport of heat, through spin fluctuations, can remain high [10] . Localization corrections associated with electron–electron interactions are also believed to induce corrections to κ e that do not scale with the WF ratio, leading to an enhancement in L / L 0 (ref. 28 ). Such interaction corrections only appear in the diffusive limit, however, below a characteristic energy scale k B T d = ћ /2 πτ determined by the impurity scattering rate 1/τ. Estimates for 1/ τ in Li 0.9 Mo 6 O 17 from in-chain resistivity or magnetoresistance measurements give T d values of order several tens of Kelvin. Whereas this estimate for the diffusion limit is consistent with the temperature ( T min ∼ 20 K) below which the resistivity starts to increase with decreasing T , the behaviour of the magnetoresistance below T min is found to be more consistent with density wave formation than localization corrections [23] . In addition, the strong violation of the WF law is observed in the metallic regime between T min and room temperature, and more significantly, above 100 K where the resistivity itself is strictly T -linear. Collectively, these observations appear to rule out localization as the origin of the WF law violation in Li 0.9 Mo 6 O 17 . Turning now to the issue of dimensionality, the form of the enhancement of the WF ratio in Li 0.9 Mo 6 O 17 is at least qualitatively consistent with the original theoretical prediction for a spinless TLL [9] . An enhancement in L xx / L 0 originates from the fact that while heat can be transmitted through a non-magnetic impurity (via spinons), the latter acts as a near-perfect reflector (back-scatterer) of charge (holons). According to this picture, L xx is predicted to be of order L 0 / K at high T , where K is the dimensionless conductance or Luttinger parameter, and as temperature is lowered, L xx / L 0 varies as a power-law, L xx / L 0 ∼ T 4−2 /K which diverges for K <0.5, corresponding to repulsive, long-range interactions [9] . Although the original model considered a single impurity embedded in an interacting spinless 1D chain, the theory has been shown to apply equally to the case of multiple impurities and the inclusion of spin degrees of freedom with only minor modifications [9] , [11] . Concerning the magnitude of the violation, a recent theoretical treatment of a weakly disordered TLL in the regime of large Umklapp scattering found an enhancement of L xx / L 0 of several orders of magnitude close to commensurate filling, owing to the fact that the spinon contribution to the thermal current cannot be degraded by Umklapp scattering processes [10] . To the best of our knowledge, no other 'gapless' model can account for such a gross violation of the WF law in the metallic regime. Although there is currently no specific theoretical framework for the thermal Hall response in a quasi-1D conductor, it has been shown theoretically that a system of weakly coupled TL chains can exhibit an electrical Hall response that shows a power-law correction to the free Fermi (band) value in the presence of Umklapp scattering [29] . Moreover, the divergence of L xy / L 0 with decreasing temperature ( Fig. 3c ) is qualitatively, if not quantitatively, similar to that found in L xx / L 0 . This divergence would seem to imply that electronic interactions in Li 0.9 Mo 6 O 17 are indeed repulsive and long range, in agreement with conclusions drawn from angle-resolved photoemission spectroscopy [19] and scanning tunnelling microscopy [20] where K , as obtained from the anomalous exponent α , is found to lie between 0.2 and 0.25. The fact that L xy / L 0 does not scale with ( L xx / L 0 ) 2 , as expected for a FL, might also be an intrinsic property of the TLL. Power-law behaviour is also predicted and indeed found in the T -dependence of the dc resistivity. Specifically, ρ b ( T ) ∼ T between 100 K and 300 K ( Fig. 1b ). The value of K extracted from the power-law exponent in ρ b ( T ) depends on the degree of commensurability. An exponent close to unity is consistent with K= 0.25 for a system at or near quarter-filling [30] . According to band-structure calculations [21] however, Li 0.9 Mo 6 O 17 is believed to be closer to half-filling, for which a T -linear resistivity corresponds to g ∼ 1 (ref. 29 ), that is, to the non-interacting case. The origin of this inconsistency is not understood at present. Since the TLL state is predicted to occur only in a strictly 1D interacting electron system, the inevitable coupling that exists between the chains in Li 0.9 Mo 6 O 17 (to generate the Hall response) and parameterized by the interchain hopping integral t ⊥ , ought to inhibit the observation of TLL physics in the zero-frequency limit [31] , [32] . (For simplicity, we assume here that t ⊥ is the same in both orthogonal directions). For k B T < t ⊥ , charge should hop coherently in all three dimensions, albeit with anisotropic velocities, and the system show characteristics of a Fermi-liquid. Once thermal broadening is comparable with the warping of the Fermi sheets, however, hopping between chains will become incoherent, leading to a putative 3D–1D dimensional crossover. Notably, in the presence of strong interactions, the value of t ⊥ can be significantly renormalized [30] , [33] and as stated above, both band structure calculations [21] and photoemission spectroscopy [19] indicate that Li 0.9 Mo 6 O 17 lies close to half-filling. Thus, provided nearest neighbour interactions are dominant, intra-chain correlation effects in Li 0.9 Mo 6 O 17 may be strong enough that its physical response is indistinguishable from that of a TLL [33] , at least at an energy scale k B T ∼ 20 K ∼ 2 meV. Below this scale, the FL ground state should recover, though whether or not such a crossover to FL physics can ever be realized in Li 0.9 Mo 6 O 17 , given its propensity to superconducting [22] and density-wave [23] order, remains to be seen. Finally, we turn to consider how one might controllably affect the interaction strength or effective dimensionality in Li 0.9 Mo 6 O 17 so that the spin and charge are recombined. One obvious route to try is to vary the band filling, for example, through substitution of Mg for Li. On the basis of the diagonal principle, the ionic radius of Li + ions is comparable with that of Mg 2+ . This suggests that such substitution could proceed without adversely affecting the 1D nature of the system, allowing the role of correlations in the TLL-to-FL crossover to be explored in a controlled manner. The results reported in this manuscript suggest that an accompanying study of the variation of L xy with doping would provide a clear litmus test of the recovery of the FL state. Sample growth and characterization Single crystals of Li 0. 9 Mo 6 O 17 were grown using a temperature gradient flux method [22] and cleaved within the a–b plane. The resulting samples were face-indexed using a single-crystal X-ray diffractometer to determine the a - and b -axes. Thereafter bar-shaped crystals (approximate dimensions 700×100×20 μm 3 ) were cut from the face-indexed sample using a wire-saw. Isolating the intrinsic in-chain resistivity To test the validity of the WF law, accurate measurements of both the electrical resistivity and thermal conductivity are essential. In a quasi-1D conductor, it is especially problematic to measure the smallest of the resistivity tensor components, because even a small admixture of either of the two larger orthogonal components can give rise to erroneous values and distort the intrinsic temperature dependence of the in-chain resistivity. In Li 0.9 Mo 6 O 17 , reported room-temperature values for the in-chain ( b axis) resistivity range from 400 μΩ cm [23] to more than 10 mΩ cm [34] , [35] . Moreover, in instances where large (that is, >1 mΩ cm) ρ b values have been reported, ρ b ( T ) tends to show a sub-linear T -dependence below 300 K. To isolate the in-chain resistivity extreme care is needed to electrically short out the sample in the two directions perpendicular to the chain and thus ensure that current flow between the voltage contacts is uniaxial. In our experiments, this is achieved either by coating conductive paint or evaporating gold strips across the entire width of the sample in the two orthogonal current directions. The mounting configuration is shown as an inset in Supplementary Figure S2 . The zero field measurements were carried out for 4.2 K < T <300 K in a 4 He dipper cryostat. In total, we measured ρ b ( T ) of over 30 single crystals to allow us to better identify the intrinsic T -dependence of the chains. For further details of how we determined the in-chain electrical resistivity, please refer to the corresponding section in the Supplementary information . Electrical Hall effect The electrical Hall effect was measured using the standard four-point method. Thin long crystals were mounted freestanding using Dupont 4929 silver epoxy. Two pairs of transverse voltage contacts were used, to check for reproducibility, and the whole process was repeated on three different samples. Owing to slight misalignment of the contacts, the measured signal contained both a symmetric (that is, magnetoresistive) and an antisymmetric part (the Hall signal). Using the relation V H =½( V ( B )− V (− B )), we were able to isolate the smaller antisymmetric Hall voltage V H , which, when normalized by B , yields the Hall coefficient R H . The uncertainty here reflects the scatter of the data from different measurements using different voltage contact pairs. To determine the Hall Lorenz number L xy (= κ xy / σ xy T ), we extract σ xy from our Hall data using the following expression: where t is the crystal thickness and I is the applied current. Thermal conductivity measurements For the thermal conductivity measurements, we used a zero-field set-up housed in a 4 He flow cryostat that covers the temperature range 10 K < T < 300 K. We employed a modified steady-state method [36] , shown schematically in Supplementary Figure S3 , in which a temperature gradient, measured using a differential thermocouple, is set up across the sample through a pair of calibrated heat-links attached to each end. The heat-links are also differential thermocouples. The sample is suspended by the free ends of the heat-links between two platforms that are weakly coupled to the heat-bath. Each platform houses a heater that enables a temperature gradient to be set up across the sample in both directions at a fixed heat-bath temperature. The thermal conductivity κ is related to the measured quantities through the relationship, where P is the power through the cross-sectional area A and l , the separation of contacts between which the temperature difference Δ T x is measured. From the temperature drop across the heat-links, we can estimate the power entering and leaving the crystal. This is a distinct advantage of the heat-link method over other thermal conductivity experimental setups, as it ensures that any power loss due to radiative losses and heat conduction through the thermocouple wires to the heat-bath is known. Although power losses due to radiation are significant (of order 20%) at high temperature, the total power loss across the sample falls to below 2% at ∼ 200 K. Provided the difference between the power entering the sample and leaving the sample remains below 20%, the power through the sample can be taken as the average of the input and output power. Regarding possible extrinsic contributions to Δ T x , thermocouple readings are always taken with and without heat input (in either current direction), and the direction of the heat current is reversed to remove any effect due to stray thermal gradients. Finally, data are always taken in the regime where the extracted value for the thermal conductivity (or thermal Hall conductivity) is independent of the strength of the heat current, thus eliminating nonlinear effects. The largest errors associated with our absolute measurement of the thermal conductivity are geometrical errors associated with the finite width of the thermocouple contacts relative to their separation, as well as with the uncertainty in determining the overall dimensions of the samples. Depending on the size of the crystal to be studied, a scanning electron, focused ion beam or high-power optical microscope was used to measure its thickness. The corresponding errors are ±1 μ m, ±1 μ m and ±5 μ m, respectively. The separation between contacts and the width of the sample was determined using a high-power optical microscope with an error of ∼ 7%. To measure the separation between contacts, we adopted the convention to measure the separation between the mid-point of the contacts for both the thermal and electrical measurements [37] . From these considerations, we associate an upper bound for the error in the final values of thermal conductivity of ±15% for the samples. The reproducibility in our measurements of κ a and κ b is shown in the Supplementary Figures S2A and S2B respectively. Thermal Hall measurements By definition, the thermal Hall effect (also known as the Righi–Leduc effect) is the development of a transverse thermal gradient (Λ T y ) in the presence of a longitudinal thermal gradient (Λ T x ) and an orthogonal magnetic field ( B z ). Crucially, Λ T x is generated by a thermal heat current along x ; J h, x =− κ xx Λ T x where κ xx is the total longitudinal thermal conductivity, including the phonon component. The transverse thermal current ( κ xy Λ T x ), due to the magnetic field deflection of the electronic charge carriers, is balanced by a heat current due to the 'total' thermal conductivity in the opposite direction. This is required by the condition that there is no net heat current flow in the transverse direction once steady state has been established. Again, inclusion of the relevant elements of the total thermal conductivity tensor leads to the following expression: giving, Hence, the thermal Hall conductivity was calculated as, where t is the thickness of the sample. To measure the thermal Hall effect, the same set-up on which the longitudinal (zero-field) thermal conductivity measurements were performed was used, although in this case, the differential thermocouple was positioned on opposite edges of the crystal. The sample was always positioned so that the heat flow in the longitudinal direction was along the b axis of the sample. The experiment was placed in an evacuated chamber immersed in liquid helium within the coil of a superconducting magnet. Heating power was provided by a resistive element thermally connected to the experimental platform and was controlled by a Lakeshore temperature controller. During a measurement of the thermal Hall effect, the temperature was first stabilized, then a fixed field applied and finally heat current passed through the sample. The modified steady state method was then employed as before. The power loss was found to be ∼ 20% at room temperature, reducing to ∼ 10% below 200 K. The experiment is then repeated at multiple field values. To isolate the thermal Hall response, both positive and negative polarities of the magnetic field were used. As with the longitudinal thermal conductivity measurements, the heat direction was then reversed and the measurements repeated. Finally, possible extrinsic contributions to the thermal Hall conductivity, for example due to anisotropy in the thermopower, are discussed in detail in the section on possible internal heating effects in the Supplementary Information . How to cite this article: Wakeham, N. et al . Gross violation of the Wiedemann–Franz law in a quasi-one-dimensional conductor. Nat. Commun. 2:396 doi: 10.1038/ncomms1406 (2011).